MicroRNA-135b promotes lung cancer metastasis by regulating multiple targets in the Hippo pathway and LZTS1 Dysregulation of microRNAs has a critical role in cancer progression. Here we identify an intronic microRNA, miR-135b that is upregulated in highly invasive non-small-cell lung cancer cells. Expression of miR-135b enhances cancer cell invasive and migratory abilities in vitro and promotes cancer metastasis in vivo , while specific inhibition of miR-135b by a miR-135b-specific molecular sponge and antagomirs suppresses cancer cell invasion, orthotopic lung tumour growth and metastasis in a mouse model. miR-135b targets multiple key components in the Hippo pathway, including LATS2, β-TrCP and NDR2, as well as LZTS1. Expression of miR-135b, LZTS1, LATS2 and nuclear TAZ predicts poor outcomes of non-small-cell lung cancer. We find that miR-135b is dually regulated by DNA demethylation and nuclear factor-kappaB signalling, implying that abnormal expression of miR-135b in cancer may result from inflammatory and epigenetic modulations. We conclude that miR-135b is an oncogenic microRNA and a potential therapeutic target for non-small-cell lung cancer. MicroRNAs (miRNAs) are a class of small, non-coding RNAs that can repress the expression of multiple target genes through the endogenous RNA interference machinery. The miRNAs can regulate a wide range of cellular functions including proliferation, apoptosis, differentiation and development [1] , [2] . Some miRNAs exert only minor effects on target gene repression, however, increasing evidence suggests that miRNAs can confer robustness of biological processes via regulation of target networks [3] , [4] . For example, miR-126 impacts endothelial recruitment by modulating the IGF1/IGF1R and GAS6/MERK pathways [5] . Recent studies have also shown that dysregulation of miRNAs is involved in carcinogenesis and metastasis in several human cancer types [6] , [7] , [8] . Lung cancers can develop a high metastatic potential, which is the major cause of treatment failure [9] . Several miRNAs, including miR-126, miR-21 and miR-335, have been associated with metastasis in several types of cancers [7] , [10] , [11] . To study the role of miRNA in lung cancer metastasis, we first established a series of lung adenocarcinoma cell sub-lines with increasing invasive and metastatic abilities [12] . We examined these sub-lines and found several miRNAs that had become deregulated in the cells with high invasive and metastatic capacity. The level of expression of miR-135b was exceptionally high among the invasion-associated miRNAs identified in these invasive cells. Previous studies have shown that miR-135b is required for osteogenic cell development [13] , and that it is enriched in the placenta where it regulates the growth rate of placental cells [14] , [15] . It has also been linked to the progression of several types of cancers [16] , [17] , [18] , and it has been found to mediate NPM-ALK-associated oncogenicity in large-cell lymphomas [19] . Although several miR-135b targets have been validated in different models [16] , [19] , the detailed mechanisms of the involvement of miR-135b or its targets in lung cancer progression remain unclear. In this study, we demonstrate that miR-135b can promote lung cancer cell invasion in vitro and metastasis in vivo . Treatment with an miR-135b sponge and an antago-135b antagomir retards tumour growth and metastasis in mouse orthotopic lung tumour models. We show that the tumour suppressor LZTS1 as well as multiple key players in the Hippo pathway, including LATS2, β-TrCP, NDR2 and TAZ, is regulated by miR-135b. In addition, we provide evidence of the potential clinical significance of miR-135b and its downstream targets in tumour specimens from non-small-cell lung cancer (NSCLC) patients. In addition, DNA methylation and inflammatory nuclear factor-kappaB (NF-κB) signalling can regulate miR-135b expression. Our results suggest that cancer cells may enact a novel dual-regulation machinery to regulate miRNA expression and promote metastatic spread by modulating a Hippo pathway network. Identification of invasion-associated miRNAs in lung cancer To identify invasion-associated miRNAs in lung cancer cells, a miRNA microarray was conducted in lung cancer cell sub-lines of increasing invasive potential [12] . Several miRNAs were found differentially expressed in these cell lines ( Supplementary Table S1 ). For example, the expression of oncomiR miR-21 was increased by approximately two-fold in highly invasive CL1-5 compared with the less invasive CL1-0 cells. In contrast, the expression of miR-126/126*, which is associated with a tumour suppressor function in invasive lung cancer cells, was decreased in CL1-5 cells [20] , [21] . The greatest elevations of miR-135b levels were found in highly invasive CL1-5 cells ( Supplementary Table S1 ). Real-time RT–PCR confirmed the expressions of miR-21, miR-126 and miR-135b in CL-series cell lines ( Fig. 1a ). In concordance with these results, miR-135b expression was positively correlated with increasing invasive activities of these lung cancer cell lines. 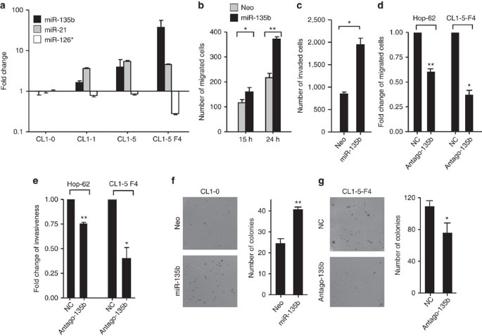Figure 1: miR-135b is upregulated in a highly invasive lung cancer cell line and modulates cell invasion and migration ability. (a) Real-time RT–PCR was conducted to quantify the endogenous expression of miR-135b, miR-21 and miR-126* in CL-series cell lines. Assays were performed in triplicate, and the results are presented as the fold-change in expression compared with CL1-0. The expression of U6B was used as a normalization control. (b) Migration assays were performed in CL1-0 cells transduced with control (Neo) or miR-135b-expressing (miR-135b) lentiviral vectors. The number of migrating cells in three different fields was counted 15 and 24 h after the inserts were removed. *P<0.05; **P<0.005 by Student’st-test. (c) An invasion assay was performed in lentiviral vector-modified CL1-0 cells as described in (b). The number of invading cells was counted 20 h after cell seeding and is presented as the mean±s.d., (d,e) CL1-5-F4 and Hop-62 cells were transfected with scramble (NC) or miR-135b-specific antagomir (Antago-135b) for 48 h and then subjected to (Fig. 1d) migration assays and (Fig. 1e) invasion assays as described above. *P<0.05; **P<0.005 by Student’st-test. (f) CL1-0 cells transduced with control (Neo) or miR-135b-expressing (miR-135b) lentiviral vectors were subjected to a soft agar assay. **P<0.005 by Student’st-test. (g) CL1-5-F4 and Hop-62 cells were transfected with the negative control (NC) or the Antago-135b for 48 h and subjected to soft agar assays. Error bars indicate mean±s.d., *P<0.05 by Student’st-test. Figure 1: miR-135b is upregulated in a highly invasive lung cancer cell line and modulates cell invasion and migration ability. ( a ) Real-time RT–PCR was conducted to quantify the endogenous expression of miR-135b, miR-21 and miR-126* in CL-series cell lines. Assays were performed in triplicate, and the results are presented as the fold-change in expression compared with CL1-0. The expression of U6B was used as a normalization control. ( b ) Migration assays were performed in CL1-0 cells transduced with control (Neo) or miR-135b-expressing (miR-135b) lentiviral vectors. The number of migrating cells in three different fields was counted 15 and 24 h after the inserts were removed. * P <0.05; ** P <0.005 by Student’s t -test. ( c ) An invasion assay was performed in lentiviral vector-modified CL1-0 cells as described in ( b ). The number of invading cells was counted 20 h after cell seeding and is presented as the mean±s.d., ( d , e ) CL1-5-F4 and Hop-62 cells were transfected with scramble (NC) or miR-135b-specific antagomir (Antago-135b) for 48 h and then subjected to ( Fig. 1d ) migration assays and ( Fig. 1e ) invasion assays as described above. * P <0.05; ** P <0.005 by Student’s t -test. ( f ) CL1-0 cells transduced with control (Neo) or miR-135b-expressing (miR-135b) lentiviral vectors were subjected to a soft agar assay. ** P <0.005 by Student’s t -test. ( g ) CL1-5-F4 and Hop-62 cells were transfected with the negative control (NC) or the Antago-135b for 48 h and subjected to soft agar assays. Error bars indicate mean±s.d., * P <0.05 by Student’s t -test. Full size image miR-135b promotes lung cancer cell growth and EMT in vitro We evaluated the effects of miR-135b on cell invasion and migration. A pri-miR-135b lentiviral expression vector was used to induce miR-135b expression in CL1-0 cells, and the miRNA levels were assayed using real-time RT–PCR ( Supplementary Fig. S1a ). The ectopic expression of miR-135b in CL1-0 cells significantly increased migratory and invasive abilities ( Fig. 1b and Supplementary Fig. S2a ). The inhibition of miR-135b by antagomiR and antisense oligonucleotides inhibited these changes in highly invasive CL1-5-F4 cells and in Hop-62 cells ( Fig. 1d , Supplementary Figs S1b, S2b ). Moreover, miR-135b promoted EMT in CL1-0 and HEK-293 cells, and inhibition of miR-135b altered the expression of E-cadherin in CL1-5 and CL141 cells ( Supplementary Fig. S3 ). Thus, the results of all of these experiments confirmed that miR-135b could promote cancer cell migration and invasion. To address other oncogenic activities modulated by miR-135b, we performed an anchorage-independent assay. Overexpression of miR-135b promoted anchorage-independent growth in CL1-0 cells ( Fig. 1f ). Conversely, miR-135b antagomir decreased the number of CL1-5-F4 cell colonies ( Fig. 1g ), suggesting that miR-135b governs both invasiveness and anchorage-independent growth in lung cancer cells. miR-135b promotes lung tumour growth and metastasis in vivo To evaluate the effect of miR-135b on tumour growth in vivo , we manipulated the expression level of miR-135b in CL1-0 cells and then performed subcutaneous xenograft of these cells into nude mice. CL1-0 cells overexpressing miR-135b exhibited enhanced tumorigenic ability 20 days after implantation ( Fig. 2a ). 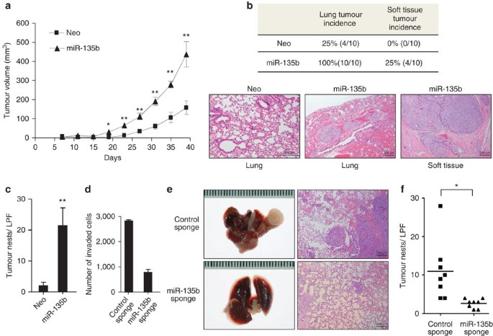Figure 2: miR-135b promotes xenograft tumour growth and metastasis in a mouse model. (a) Nude mice were subcutaneously injected with 1.2 × 106CL1-0 cells that stably expressed either control vector (Neo) or miR-135b lentiviral vectors. After implantation for 7 days, tumour volume measurement began and was performed every 4 days.(n=9) Mean±s.e.m., *P<0.05, **P<0.005 by Student’st-test. (b,c) CL1-0 cells that were transduced with control (Neo) or miR-135b-expressing lentiviral vectors were intravenously injected into NOD-SCID mice (10 mice per group). (b) The statistical incidence of lung or soft tissue tumour generation in the mice after injection with CL1-0 cells with different vector-transduced cells. The animals were killed 8 weeks after injection, and lung sections were examined by hematoxylin/eosin (H&E) staining. Scale bar, 200 μm. (c) The number of lung tumour nests in each group was counted under a low power field (LPF) and is presented as the mean±s.d., **P<0.005 by Student’st-test. (d) CL1-5-F4 cells transfected with plasmids expressing either control or miR-135b sponges were analysed using anin vitroinvasion assay. The average number of invading cells obtained in the transwell invasion assay is presented (n=3). (e,f) CL1-5-F4 cells stably expressing control sponge or miR-135b sponge were intravenously injected into SCID mice (n=8). Representative pictures of murine whole lung (left) and H&E staining of lung sections (right) are presented. (f) Lung tumour nests in each group were examined and counted using a microscope (n=8). Mean±s.e.m. is shown, *P<0.05 by Student’st-test. Figure 2: miR-135b promotes xenograft tumour growth and metastasis in a mouse model. ( a ) Nude mice were subcutaneously injected with 1.2 × 10 6 CL1-0 cells that stably expressed either control vector (Neo) or miR-135b lentiviral vectors. After implantation for 7 days, tumour volume measurement began and was performed every 4 days. ( n =9) Mean±s.e.m., * P <0.05, ** P <0.005 by Student’s t -test. ( b , c ) CL1-0 cells that were transduced with control (Neo) or miR-135b-expressing lentiviral vectors were intravenously injected into NOD-SCID mice (10 mice per group). ( b ) The statistical incidence of lung or soft tissue tumour generation in the mice after injection with CL1-0 cells with different vector-transduced cells. The animals were killed 8 weeks after injection, and lung sections were examined by hematoxylin/eosin (H&E) staining. Scale bar, 200 μm. ( c ) The number of lung tumour nests in each group was counted under a low power field (LPF) and is presented as the mean±s.d., ** P <0.005 by Student’s t -test. ( d ) CL1-5-F4 cells transfected with plasmids expressing either control or miR-135b sponges were analysed using an in vitro invasion assay. The average number of invading cells obtained in the transwell invasion assay is presented ( n =3). ( e , f ) CL1-5-F4 cells stably expressing control sponge or miR-135b sponge were intravenously injected into SCID mice ( n =8). Representative pictures of murine whole lung (left) and H&E staining of lung sections (right) are presented. ( f ) Lung tumour nests in each group were examined and counted using a microscope ( n =8). Mean±s.e.m. is shown, * P <0.05 by Student’s t -test. Full size image To test the effects of miR-135b on in vivo cell metastasis, we stably transduced CL1-0 cells with a miR-135b-expressing lentiviral vector. NOD-SCID mice were intravenously injected with CL1-0 cells and sacrificed after 8 weeks. miR-135b expression promoted metastasis in lung and soft tissues ( Fig. 2b ). Furthermore, we investigated whether suppression of miR-135b expression would impede lung cancer invasion and metastasis. A miR-135-specific sponge carrying seven repeats of the miR-135b binding site was constructed to neutralize endogenous miR-135b activity [22] . Highly invasive CL1-5-F4 cells stably expressing either a control or the miR-135b sponge were analysed by transwell invasion assay, and cells expressing the miR-135b sponge diminished the invasive activity ( Fig. 2d ). Next, we intravenously injected the SCID mice with control or miR-135b sponge-producing CL1-5-F4 cells and counted the number of metastatic lung nodules 6 weeks later ( Fig. 2e ). The number of tumour nodules that developed in the mouse lungs was significantly reduced in the miR-135b sponge group ( P =0.0126) ( Fig. 2f ). The overexpression of miR-135b in highly invasive cells appeared to be required for in vivo lung cancer growth and metastasis in these experiments. miR-135b antagomir inhibits lung tumour growth and metastasis We examined the therapeutic potential of miR-135b antagomir in three sets of animal models. First, we tested the effects of the inhibition of endogenous miR-135b on tumour growth in xenograft tumours. The growth of H441 human lung adenocarcinoma cells, which express high levels of endogenous miR-135b ( Supplementary Fig. S4 ), was inhibited when antago-135b antagomir was administered before xenograft implantation. This inhibitory activity was sustained when miR-135b antagomir was systematically injected 4 days after cancer cell implantation, ( Supplementary Fig. S14 ) and we found that the incidence and volume were significantly reduced in the xenograft tumours ( Fig. 3a ). 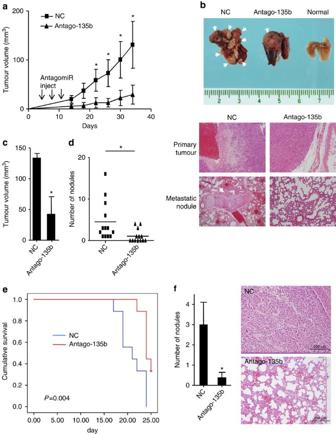Figure 3: Systemic delivery of antagomiR-135b inhibits metastasis and tumour growthin vivo. (a) Nude mice were subcutaneously injected with 5 × 105H441 cells. Scramble antagomir (NC) or miR-135b Antagomir (antago-135b) was administered via tail vein injection 2 days after implantation. On day 14 after cancer cell implantation, tumour volume measurements began and were performed every 4 days (n=9). Mean±s.e.m. is shown, *P<0.05 by Student’st-test; (b–d) CL1-5 cells were implanted orthotopically into the left lungs of 6-week-old nude mice (n=9). A series of scramble antagomir (NC) or miR-135b antagomir (Antago-135b) intravenous injections were performed every 2 days after tumour cell implantation. Lungs were harvested 25 days after the cells were implanted. (b) Bright-field imaging and H&E staining of CL1-5 tumour-bearing lungs. Arrows indicate the visible nodules. (c) Primary tumour volume and (d) number of intra-lung metastatic nodules in CL1-5 tumour-bearing mice treated with scramble antagomir (NC) or miR-135b antagomir (Antago-135b) 25 days after orthotopic implantation. Data are expressed as the mean±s.e.m. *P<0.05 by Student’st-test. (e) Mice bearing CL1-5 cells were subjected to scramble antagomir (NC) or miR-135b antagomir (Antago-135b) treatment. Animal survival was determined using Kaplan–Meier analysis and the log-rank test for data obtained 25 days after the cancer cells were orthotopically injected. (n=9) (f) CL1-5-F4 cells with scramble antagomir (NC) or miR-135b antagomir (Antago-135b) were intravenously injected to assess the effect of antagomir on late-stage metastasis. (n=9). Representative average of visible metastatic lung nodules and H&E staining (right). Data are expressed as the mean±s.e.m. *P<0.05 by Student’st-test. Figure 3: Systemic delivery of antagomiR-135b inhibits metastasis and tumour growth in vivo . ( a ) Nude mice were subcutaneously injected with 5 × 10 5 H441 cells. Scramble antagomir (NC) or miR-135b Antagomir (antago-135b) was administered via tail vein injection 2 days after implantation. On day 14 after cancer cell implantation, tumour volume measurements began and were performed every 4 days ( n =9). Mean±s.e.m. is shown, * P <0.05 by Student’s t -test; ( b–d ) CL1-5 cells were implanted orthotopically into the left lungs of 6-week-old nude mice ( n =9). A series of scramble antagomir (NC) or miR-135b antagomir (Antago-135b) intravenous injections were performed every 2 days after tumour cell implantation. Lungs were harvested 25 days after the cells were implanted. ( b ) Bright-field imaging and H&E staining of CL1-5 tumour-bearing lungs. Arrows indicate the visible nodules. ( c ) Primary tumour volume and ( d ) number of intra-lung metastatic nodules in CL1-5 tumour-bearing mice treated with scramble antagomir (NC) or miR-135b antagomir (Antago-135b) 25 days after orthotopic implantation. Data are expressed as the mean±s.e.m. * P <0.05 by Student’s t -test. ( e ) Mice bearing CL1-5 cells were subjected to scramble antagomir (NC) or miR-135b antagomir (Antago-135b) treatment. Animal survival was determined using Kaplan–Meier analysis and the log-rank test for data obtained 25 days after the cancer cells were orthotopically injected. ( n =9) ( f ) CL1-5-F4 cells with scramble antagomir (NC) or miR-135b antagomir (Antago-135b) were intravenously injected to assess the effect of antagomir on late-stage metastasis. ( n =9). Representative average of visible metastatic lung nodules and H&E staining (right). Data are expressed as the mean±s.e.m. * P <0.05 by Student’s t -test. Full size image Next, we checked the effects of miR-135b inhibition on tumour growth and metastasis in an orthotopic lung cancer model. Seven intravenous injections of miR-135b antagomir were given 4 days after CL1-5 implantation. Compared with the control lungs, miR-135b antagomir inhibited orthotopic tumour growth ( Fig. 3b ) and decreased the volume of lung metastases ( Fig. 3b ). In addition, even though the severe growth of orthotopic tumours caused cachexia and death of the mice, systemic delivery of the antago-135b antagomir in the tumour-bearing mice increased survival rates ( Fig. 3e ). We further determined the impact of the antagomir during the late stages in metastasis, such as extravasation and colonization. Intravenous injections of highly invasive CL1-5-F4 cells in the mice were followed by a succession of either control- or antago-135b treatments via the tail vein. On evaluation 3 months after the cells were injected, the antago-135b-treated group had generated eight-fold fewer metastatic lung nodules than the control group ( Fig. 3f ; P =0.018). Thus, with miR-135b as a therapeutic target, the administration of antago-135 antagomir controlled lung cancer growth and metastasis in the experimental mouse models. miR-135b regulates LZTS1 and control cancer invasion We used the computational algorithms of TargetScan (Version 5.2) [23] for prediction analysis to identify target genes of miR-135b. Several candidates were discovered, and their 3′-UTRs (3′-untranslated regions) were conjugated with luciferase for reporter assays. LZTS1 has the potential to suppress the invasion and motility of melanoma cells [24] , and its expression is associated with lymph node metastasis in breast cancer patients [25] . In our experiments, the luciferase activity of plasmids containing the 3′-UTR of LZTS1 was significantly reduced in the presence of miR-135b ( Fig. 4a and Supplementary Fig. S5 ). The putative miR-135b seed sequence mutations were introduced to further investigate the direct regulatory effect. The reporter assay showed that the effects of miR-135b repression were abolished when both putative seed sequences were mutated ( Fig. 4b and Supplementary Fig. S5 ). The suppressive effects of miR-135b on the LZTS1 3′-UTR-carrying luciferase were significantly reduced by the antago-135 antagomir ( Fig. 4c ). These results indicated that miR-135b regulated the expression of LZTS1 through a direct seed sequence interaction. 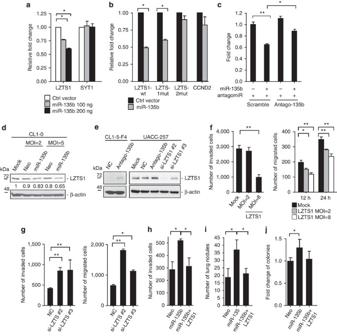Figure 4: LZTS1 is a direct target of miR-135b. (a) Co-transduction of CL1-0 cells with a control vector (Ctrl vector) or a miR-135b-expressing plasmid with firefly luciferase fused with 3′-UTR sequences of putative miR-135b target genes. Luciferase activity was measured, and the relative ratio of the activity in the miR-135b groups to that in the control vector group is presented as the mean±s.d., *P<0.05 by Student’st-test. (b) CL1-0 cells were co-transfected with Ctrl vector- or miR-135b-expressing plasmids and firefly luciferase fused with wild-type (wt) LZTS1 3′-UTR or seed sequence-mutated (mut) 3′-UTR (1mut, seed 1 mutated; 2mut, both seeds mutated). Mean±s.d. is shown, *P<0.05 by Student’st-test. (c) CL1-0 cells were co-transfected with miR-135b, wild-type LZTS1 3′-UTR along with Scramble or miR-135b-specific antagomir (Antago-135b). Luciferase activity was measured and is presented as described in (a). Mean±s.d. is shown, *P<0.05; **P<0.005 by Student’st-test. (d) Western blot analysis of endogenous LZTS1 expression in CL1-0 cells after transduction with different multiplicities of infections of control (Neo) or miR-135b-expressing lentiviral vectors. (e) CL1-5-F4 and UACC-257 cells were administered with 100 nM of negative control (NC) or antago-135b for 48 h. Total cell lysates were harvested for western blot analysis. (f) The cells were transduced with different amounts of LZTS1-expressing lentiviral vector, and western blot analysis of LZTS1 expression along with analyses of invasion and migration ability were conducted as described above. Mean±s.d. is shown, *P<0.05; **P<0.005 by Student’st-test. (g) UACC-257 cells were transfected with control (NC) or LZTS1-specific siRNAs (si-LZTS1 no. 2 and no. 3) for 48 h and subjected to invasion and migration assays as described above. Mean±s.d. is shown, *P<0.05; **P<0.005 by Student’st-test. (h) CL1-0 cells stably expressing control vector, miR-135b or co-expressing miR-135b and LZTS1 were analysed in transwell invasion assays. Mean±s.d. is shown, *P<0.05 by Student’st-test. (i) The statistical incidence of lung nodule generation in the mice after injecting CL1-0 cells with different vector-transduced cells. The animals were killed 8 weeks after injection(n=6). Mean±s.e.m. is shown, *P<0.05 by Student’st-test. (j) The number of colonies of soft agar assay by CL1-0 cell derivatives with Neo-control, miR-135b or miR-135b+ LZTS1 (n=3). Mean±s.d. is shown, *P<0.05 by Student’st-test. Figure 4: LZTS1 is a direct target of miR-135b. ( a ) Co-transduction of CL1-0 cells with a control vector (Ctrl vector) or a miR-135b-expressing plasmid with firefly luciferase fused with 3′-UTR sequences of putative miR-135b target genes. Luciferase activity was measured, and the relative ratio of the activity in the miR-135b groups to that in the control vector group is presented as the mean±s.d., * P <0.05 by Student’s t -test. ( b ) CL1-0 cells were co-transfected with Ctrl vector- or miR-135b-expressing plasmids and firefly luciferase fused with wild-type (wt) LZTS1 3′-UTR or seed sequence-mutated (mut) 3′-UTR (1mut, seed 1 mutated; 2mut, both seeds mutated). Mean±s.d. is shown, * P <0.05 by Student’s t -test. ( c ) CL1-0 cells were co-transfected with miR-135b, wild-type LZTS1 3′-UTR along with Scramble or miR-135b-specific antagomir (Antago-135b). Luciferase activity was measured and is presented as described in ( a ). Mean±s.d. is shown, * P <0.05; ** P <0.005 by Student’s t -test. ( d ) Western blot analysis of endogenous LZTS1 expression in CL1-0 cells after transduction with different multiplicities of infections of control (Neo) or miR-135b-expressing lentiviral vectors. ( e ) CL1-5-F4 and UACC-257 cells were administered with 100 nM of negative control (NC) or antago-135b for 48 h. Total cell lysates were harvested for western blot analysis. ( f ) The cells were transduced with different amounts of LZTS1-expressing lentiviral vector, and western blot analysis of LZTS1 expression along with analyses of invasion and migration ability were conducted as described above. Mean±s.d. is shown, * P <0.05; ** P <0.005 by Student’s t -test. ( g ) UACC-257 cells were transfected with control (NC) or LZTS1-specific siRNAs (si-LZTS1 no. 2 and no. 3) for 48 h and subjected to invasion and migration assays as described above. Mean±s.d. is shown, * P <0.05; ** P <0.005 by Student’s t -test. ( h ) CL1-0 cells stably expressing control vector, miR-135b or co-expressing miR-135b and LZTS1 were analysed in transwell invasion assays. Mean±s.d. is shown, * P <0.05 by Student’s t -test. ( i ) The statistical incidence of lung nodule generation in the mice after injecting CL1-0 cells with different vector-transduced cells. The animals were killed 8 weeks after injection( n =6). Mean±s.e.m. is shown, * P <0.05 by Student’s t -test. ( j ) The number of colonies of soft agar assay by CL1-0 cell derivatives with Neo-control, miR-135b or miR-135b+ LZTS1 ( n =3). Mean±s.d. is shown, * P <0.05 by Student’s t -test. Full size image Next, the luciferase gene was replaced by the LZTS1 coding sequence to mimic the endogenous LZTS1 transcript. The overexpression of miR-135b decreased the expression of HA-tagged LZTS1 protein in a dose-dependent manner ( Supplementary Fig. S6 ). The miR-135b-mediated suppression was negated by mutation of the miR-135b seed sequences on the LZTS1 3′-UTR ( Supplementary Fig. S6 ). To investigate whether miR-135b regulates endogenous LZTS1, the expression of LZTS1 in miR-135b-expressing lentiviral vector-transduced cells was evaluated. As shown in Fig. 4d , endogenous LZTS1 expression in the lung cancer cell line CL1-0 was decreased by the ectopic expression of miR-135b ( Fig. 4d ). The same phenomenon was observed in UACC-257 melanoma cells and in MDA-MB-435 cells ( Supplementary Fig. S7 ). In contrast, blocking of miR-135b with antisense oligonucleotides significantly increased LZTS1 expression in CL1-5-F4 and UACC-257 cells ( Fig. 4e ). These results demonstrated that miR-135b-mediated LZTS1 repression is possible in lung cancer cells and in other types of cancer cells. To explore the biological function of LZTS1 in lung cancer cells, a lentiviral vector containing the complete coding sequence of LZTS1 was transduced into A549 cells ( Supplementary Fig. S8 ). The ectopic expression of LZTS1 suppressed cell invasion and migration in a dose-dependent manner ( Fig. 4f ), while suppression of LZTS1 expression by double-strand siRNA in UACC-257 cells enhanced cell invasion and migration ( Fig. 4g ). This resembled the effects of miR-135b overexpression in low-invasive cells. Conversely, the invasive activity was reduced if miR-135b was overexpressed in conjunction with LZTS1 in CL1-0 cells ( Fig. 4h ). The in vivo metastatic assay also showed that LZTS1 remarkably suppressed the lung metastatic nodules and was sufficient to repress miR-135b-dependent metastatic colonization and Slug ( Fig. 4i and Supplementary Fig. S9 ). However, an overexpression of LZTS1 in miR-135b-expressing cells did not repress the miR-135b-driven colony-forming activity ( Fig. 4j ). These results suggest that the major function of the miR-135b-LZTS1 axis in lung cancer is the suppression of cancer metastasis. miR-135b regulates multiple components of Hippo pathway The Hippo pathway has an important role in controlling organ size in Drosophila melanogaster and tumorigenesis in mammals. The central axis of the Hippo pathway is a kinase cascade that includes MST1, LATS1/2 (serine/threonine-protein kinase 1/2) and MOB1a/b (Mob kinase activator 1a/b), along with downstream TAZ oncogenic effectors [26] . Phosphorylation of TAZ is initiated at Ser 311, and CK1 phosphorylates Ser 314, which leads to a SCF β-TrCP (beta-transducin repeat-containing protein)-mediated ubiquitination and degradation [27] . NDR1/2 (nuclear Dbf2-related kinase 1/2) and FOXO1 are also phosphorylated by MST1 when the Hippo pathway is activated, and this is thought to assist with the tumour suppressive function of MST1 (ref. 28 ). Based on a TargetScan (Version 5.2) prediction, six Hippo pathway-related genes were identified to contain putative miR-135b target sites on their 3′-UTRs ( Supplementary Fig. S10 ). In agreement with this, a negative correlation between endogenous LATS2 and TAZ expressions in CL-series cells was observed ( Supplementary Fig. S11 ). The results of a luciferase reporter assay showed that miR-135b could downregulate the canonical Hippo pathway protein LATS2 as well parallel molecules including β-TrCP, NDR2 and MOB1b ( Fig. 5a ). Administration of the antago-135b antagomir resulted in a decrease in miR-135b-induced reporter activity ( Fig. 5b ). Endogenous protein levels of LATS2, β-TrCP and NDR2 were downregulated in miR-135b-expressing CL1-0 and HEK-293 cells ( Fig. 5c ). Conversely, TAZ, a major Hippo downstream effector, was upregulated in the miR-135b-overexpressing cells ( Fig. 5c and Supplementary Fig. S12a ). 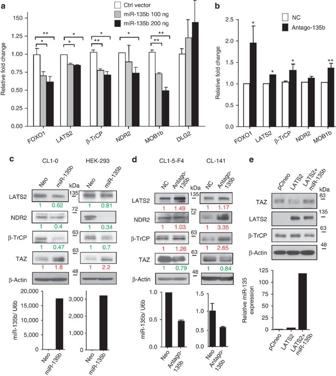Figure 5: Multiple components of a Hippo pathway are regulated by miR-135b. (a) CL1-0 cells were co-transfected with control vector (Ctrl vector) or miR-135b-expressing plasmids with firefly luciferase fused with 3′-UTR sequences of putative miR-135b target genes. Luciferase activity was measured, and the relative ratio of activity in the miR-135b groups to that in the control vector groups is presented as the mean±s.d., *P<0.05; **P<0.01 by Student’st-test. (b) CL1-0 cells co-transfected with miR-135b and pGL3-3′-UTRs with scramble (NC) or Antago-135b for 60 h. Luciferase activity was assayed and is presented as described in (a). Mean±s.d. is shown, *P<0.05; **P<0.005 by Student’st-test. (c) Western blot analysis of the Hippo pathway components in CL1-0 and HEK-293 cells transduced with control (Neo) or miR-135b lentiviral vectors. (d) Western blot analysis of Hippo pathway proteins in CL1-5-F4 and CL-141 cells incubated with Scramble (NC) or Antago-135b for 72 h. Quantitative RT–PCR was used to assay miR-135b knockdown activity. (e) Endogenous TAZ proteins in CL1-0 cells transfected with control (pCIneo), miR-135b, miR-135+ LATS2. The cells were harvested after 36 h of transfection. Figure 5: Multiple components of a Hippo pathway are regulated by miR-135b. ( a ) CL1-0 cells were co-transfected with control vector (Ctrl vector) or miR-135b-expressing plasmids with firefly luciferase fused with 3′-UTR sequences of putative miR-135b target genes. Luciferase activity was measured, and the relative ratio of activity in the miR-135b groups to that in the control vector groups is presented as the mean±s.d., * P <0.05; ** P <0.01 by Student’s t -test. ( b ) CL1-0 cells co-transfected with miR-135b and pGL3-3′-UTRs with scramble (NC) or Antago-135b for 60 h. Luciferase activity was assayed and is presented as described in ( a ). Mean±s.d. is shown, * P <0.05; ** P <0.005 by Student’s t -test. ( c ) Western blot analysis of the Hippo pathway components in CL1-0 and HEK-293 cells transduced with control (Neo) or miR-135b lentiviral vectors. ( d ) Western blot analysis of Hippo pathway proteins in CL1-5-F4 and CL-141 cells incubated with Scramble (NC) or Antago-135b for 72 h. Quantitative RT–PCR was used to assay miR-135b knockdown activity. ( e ) Endogenous TAZ proteins in CL1-0 cells transfected with control (pCIneo), miR-135b, miR-135+ LATS2. The cells were harvested after 36 h of transfection. Full size image We also confirmed regulation of the Hippo pathway by miR-135b by treatment of CL1-5-F4 and CL141 cells with the antago-135b antagomir. Inhibition of miR-135b reduced TAZ protein expression and induced LATS2, β-TrCP and NDR2 expressions, and endogenous TAZ was downregulated in miR-135b suppressed lung cancer cell lines ( Fig. 5d and Supplementary Fig. S12b ). To further determine whether the canonical Hippo components were epistatically regulated by miR-135b, we explored the function of miR-135b and the Hippo downstream effector, TAZ. Transient expression of LATS2 in CL1-5 cells decreased the TAZ protein level ( Fig. 5e ). However, when miR-135b was introduced the endogenous TAZ was recovered, indicating that the expression of TAZ was associated with miR-135b ( Fig. 5e ). We further identified the functions of the Hippo component, LATS2, and its downstream effector TAZ. Although ectopic LATS2 did not affect cancer cell migration, invasion and colony-forming activity ( Supplementary Fig. S13a,b ), knockdown of TAZ dramatically reduced cancer cell invasive and colony-forming abilities ( Supplementary Fig. S13c ). These findings suggest that miR-135b contributes to the oncogenic activation of TAZ via multiple targets in a Hippo pathway. Clinical correlations of miR-135b and its targets in NSCLC To further understand the potential biological significance of deregulated miR-135b expression in lung cancer progression, we evaluated the correlation of the miR-135b expression profile with overall survival in tumour specimens from 112 lung cancer patients ( Supplementary Table S2 ). miR-135b levels were measured by real-time RT–PCR, and Kaplan–Meier analysis showed that high levels of miR-135b expression were significantly associated with decreased overall survival ( P =0.0019; Fig. 6a ). Cox proportional hazard regression analysis with a stepwise selection model also demonstrated that the overall survival of this cohort was correlated with the miR-135b expression levels (HR=2.24) ( Supplementary Table S3 ). 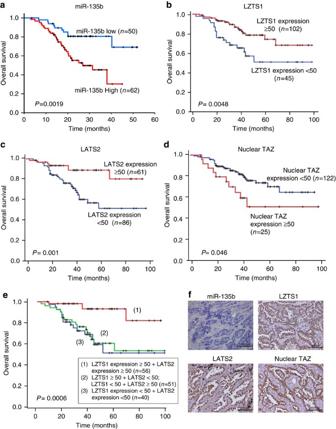Figure 6: Kaplan–Meier analysis of NSCLC patients with different expression levels of miR-135b and its targets. (a) Kaplan–Meier plots of overall survival in 112 NSCLC patients in high- and low-risk groups based on miR-135b expression levels. (b–e) Expressions of LZTS1, LATS2 and TAZ proteins were examined via immunohistochemical staining in serial dissections of primary tumour specimens from 147 NSCLC patients who underwent surgical resections. Patients were designated as having high LZTS1 or LATS2 expression if more than 50% of the neoplastic cells in the tumour sections had positive immunoreactivity, and as having low LZTS1 or LATS2 expression if fewer than 50% of the cells were immunoreactive (b,c). The patients were designated as having high nuclear TAZ expression if more than 50% of the neoplastic cells had a positive TAZ signal in the nucleus, and as having low nuclear TAZ expression if fewer than 50% of the neoplastic cells had a positive TAZ signal in the nucleus (d). The results shown reflect Kaplan–Meier estimates of overall survival for NSCLC patients according to their expression levels of LZTS1 (b), LATS2 (c), nuclear TAZ (d) and both LZTS1 and LATS2 (e).P-values were obtained from two-sided log-rank tests (f).In situhybridization of miR-135b (upper panel) and immunohistochemical analysis of LZTS1 (lower panels) expression in serial sections of NSCLC tumor specimens. scale bar: 100μm. Figure 6: Kaplan–Meier analysis of NSCLC patients with different expression levels of miR-135b and its targets. ( a ) Kaplan–Meier plots of overall survival in 112 NSCLC patients in high- and low-risk groups based on miR-135b expression levels. ( b – e ) Expressions of LZTS1, LATS2 and TAZ proteins were examined via immunohistochemical staining in serial dissections of primary tumour specimens from 147 NSCLC patients who underwent surgical resections. Patients were designated as having high LZTS1 or LATS2 expression if more than 50% of the neoplastic cells in the tumour sections had positive immunoreactivity, and as having low LZTS1 or LATS2 expression if fewer than 50% of the cells were immunoreactive ( b , c ). The patients were designated as having high nuclear TAZ expression if more than 50% of the neoplastic cells had a positive TAZ signal in the nucleus, and as having low nuclear TAZ expression if fewer than 50% of the neoplastic cells had a positive TAZ signal in the nucleus ( d ). The results shown reflect Kaplan–Meier estimates of overall survival for NSCLC patients according to their expression levels of LZTS1 ( b ), LATS2 ( c ), nuclear TAZ ( d ) and both LZTS1 and LATS2 ( e ). P -values were obtained from two-sided log-rank tests ( f ). In situ hybridization of miR-135b (upper panel) and immunohistochemical analysis of LZTS1 (lower panels) expression in serial sections of NSCLC tumor specimens. scale bar: 100μm. Full size image We next examined the expression of the miR-135b downstream target genes, LZTS1 and LATS2, as well as nuclear TAZ, by immunohistochemical analysis of 147 NSCLC tumour samples ( Supplementary Table S4 ). Kaplan–Meier and log-rank test analyses demonstrated that lower LZTS1 expressions were associated with poor overall survival ( P =0.048; Fig. 6b ). In addition, we observed inverse correlations with miR-135b expression levels by in situ hybridization and LZTS1 protein levels by immunohistochemistry in the same tumour sections ( Supplementary Fig. S15 ). Tumour specimens with a low expression of LATS2 were associated with poorer overall survival ( P =0.0015; Fig. 6c ). Multivariate Cox analysis demonstrated that both LZTS1 (HR=0.494, 95% CI=0.251 to 0.971; P =0.0409) and LATS2 (HR=0.416, 95% CI=0.176 to 0.983; P =0.0455) were protective factors when age, gender and tumour histological type were considered ( Supplementary Table S5 ), which suggests that patients with tumours expressing higher levels of LZTS1 or LATS2 may have a lower risk of mortality. In addition, nuclear TAZ was found to be a risk factor for survival outcome (HR=3.079, 95% CI=1.409 to 6.727; P =0.0048). High levels of nuclear TAZ staining, which indicated TAZ activation in the tumour specimens, were associated with poor overall survival in the patients ( P =0.049; Fig. 6d ). When we further analysed the combined effects of both proteins on the prognosis of NSCLC patients, we found that patients with tumours expressing higher levels of LZTS1 and LATS2 had better overall survival than those whose tumours showed low LZTS1 and LATS2 expressions ( P =0.0006; Fig. 6e ). Multivariate Cox analysis also showed that these two proteins were protective factors if both were expressed at higher levels (HR=0.575, 95% CI=0.368 to 0.898; P =0.0149). These results indicated that the survival of NSCLC patients strongly associated with miR-135b and its LZTS1 and LATS2 targets. Fig. 6f shows a typical in situ hybridization signal of miR-135b and immunohistochemical staining of LZTS1, LATS2 and nuclear TAZ. The expressions of miR-135b, LZTS1, LATS2 and nuclear TAZ may therefore be a useful prognostic signature for NSCLC. Dual transcriptional regulation of miR-135b expression Based on the above results, miR-135b was identified as an invasion/metastasis modulator. In order to elucidate the mechanism underlying the deregulation of miR-135b, we used differential methylation hybridization (DMH) microarray screening and found that the promoter region of miR-135b was hypomethylated in CL1-5 cells compared with the same region in normal human bronchial epithelial and CL1-0 cells ( Supplementary Fig. S16 ). Corresponding to the results of the DMH array, there was a putative CpG island in the miR-135b promoter region [29] ( Supplementary Fig. S17a ). We further verified the DMH array results in CL-series lung cancer cell lines. Bisulfite sequencing and quantitative methylation-specific PCR (qMS-PCR) of the miR-135b CpG island region confirmed that the methylation levels of the miR-135b promoter regions were lower in the highly invasive lung cancer cell lines ( Fig. 7a ). Moreover, the miR-135b expression levels in the cancer cells were restored by the DNA methylation inhibitor 5-aza-2′-CdR ( Fig. 7c ). 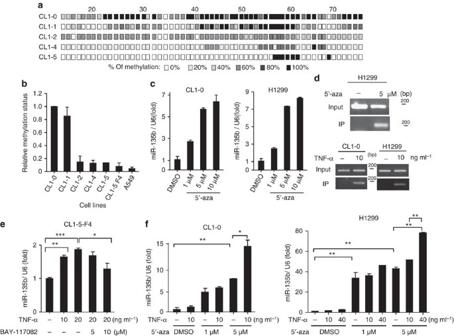Figure 7: Dual regulations of the expression of miR-135b by DNA demethylation and NF-κB signalling. (a) Bisulfite sequencing analysis was performed in CL-series cells. Each square represents a CpG dinucleotide, and the colours indicate the percentage of methylation. (b) Quantitative methylation-specific PCR (qMS-PCR) was performed to analyse the amount of methylated (M) and unmethylated (U) DNA in CL-series cells. The ratio of M to U in each cell line was calculated and is presented as the mean±s.d. of the ratios compared with the M to U ratio in CL1-0 cells. (c) Cells were treated with different doses of 5-aza-2′-CdR (5-aza) for 4 days, and total RNA was harvested for real-time RT–PCR. Data are expressed as the mean±s.d., (d) The cells were treated with the indicated amounts of 5-aza-2′-CdR (upper panel) for 4 days or TNF-α (lower panel) for 6 h before being subjected to chromatin immunoprecipitation (ChIP) with anti-p65 antibody and specific primers. (e) CL1-5-F4 cells were treated with different concentrations of TNF-α with or without BAY-117082 (5 or 10 μM) for 6 h. Total RNA was harvested, and miR-135b expression was analysed and analysis by real-time RT–PCR. Mean±s.d. is shown. *P<0.05; **P<0.00, ***P<0.001 by Student’st-test. (f) Cells were treated with or without 5-aza-2′-CdR for 4 days and re-seeded for TNF-α stimulation for 6 h. Total RNA was harvested, and miR-135b expression was analysed. Mean±s.d. is shown, *P<0.05; **P<0.005 by Student’st-test. Figure 7: Dual regulations of the expression of miR-135b by DNA demethylation and NF-κB signalling. ( a ) Bisulfite sequencing analysis was performed in CL-series cells. Each square represents a CpG dinucleotide, and the colours indicate the percentage of methylation. ( b ) Quantitative methylation-specific PCR (qMS-PCR) was performed to analyse the amount of methylated (M) and unmethylated (U) DNA in CL-series cells. The ratio of M to U in each cell line was calculated and is presented as the mean±s.d. of the ratios compared with the M to U ratio in CL1-0 cells. ( c ) Cells were treated with different doses of 5-aza-2′-CdR (5-aza) for 4 days, and total RNA was harvested for real-time RT–PCR. Data are expressed as the mean±s.d., ( d ) The cells were treated with the indicated amounts of 5-aza-2′-CdR (upper panel) for 4 days or TNF-α (lower panel) for 6 h before being subjected to chromatin immunoprecipitation (ChIP) with anti-p65 antibody and specific primers. ( e ) CL1-5-F4 cells were treated with different concentrations of TNF-α with or without BAY-117082 (5 or 10 μM) for 6 h. Total RNA was harvested, and miR-135b expression was analysed and analysis by real-time RT–PCR. Mean±s.d. is shown. * P <0.05; ** P <0.00, *** P <0.001 by Student’s t -test. ( f ) Cells were treated with or without 5-aza-2′-CdR for 4 days and re-seeded for TNF-α stimulation for 6 h. Total RNA was harvested, and miR-135b expression was analysed. Mean±s.d. is shown, * P <0.05; ** P <0.005 by Student’s t -test. Full size image miR-135b is an intronic miRNA located in the intron 1 region of LEMD1 . We hypothesized that expressions of both genes were driven by the same promoter. The expression levels of miR-135b and LEMD1 in lung cancer cell lines were similar ( Supplementary Fig. S17b ). Additionally, 5-aza-2′-CdR treatment restored LEMD1 mRNA expression in a dose-dependent manner ( Supplementary Fig. S17c ). Taken together, these results indicated that the promoter region of miR-135b can be epigenetically regulated by DNA methylation in lung cancer cells. In addition to the DNA methylation results, we also found a putative NF-κB-binding site in the CpG island in the miR-135b promoter region ( Supplementary Fig. S17a , predicted by http://www.cbrc.jp/research/db/TFSEARCH.html ). Thus, we examined the effect of NF-κB activation on miR-135b expression by chromatin immunoprecipitation assay. The putative NF-κB binding site within the miR-135b promoter was occupied by p65 when CL1-0 cells were treated with 5-aza-2′-CdR ( Fig. 7d , upper panel). When we used TNF-α to stimulate NF-κB activation, the association of NF-κB with the miR-135b promoter was confirmed ( Fig. 7d , lower panel). The effect of NF-κB signalling-induced miR-135b expression was also observed in H1299 and CL1-5-F4 cells after treatment with TNF-α( Fig. 7e and Supplementary Fig. S18 ). The TNF-α-stimulated miR-135b expression was negated by a NF-κB inhibitor BAY-117082, further supporting the role NF-κB activation in mediating the upregulation of miR-135b ( Fig. 7e and Supplementary Fig. S18 ). Thus, DNA methylation may prohibit the binding of the NF-κB transactivation complex to the miR-135b promoter region. To evaluate this possibility, we measured methylation levels of the 10 GpC regions in the NF-κB binding sites of the miR-135b promoter region using a quantitative pyrosequencing assay ( Supplementary Fig. S19a ). The results revealed that the percentage of methylation of the CpG sites of putative NF-κB binding sites in CL1-0 and CL1-1 cells were higher than in CL1-5 and CL1-5-F4 cells ( Supplementary Fig. S19b,c ), which implied that DNA methylation hindered NF-κB-miR-135b binding. To clarify whether DNA methylation and NF-κB worked together to regulate miR-135b transcription, CL1-0 and H1299 cells were co-treated with 5-aza-2′-CdR and TNF-α. The expression of miR-135b was dramatically elevated compared with the expression resulting from a single treatment by either molecule alone ( Fig. 7f ), whereas LATS2 and LZTS1 were gradually decreased in the H1299 cells ( Supplementary Fig. S20 ), suggesting that miR-135b and its targets are synergistically regulated by these two mechanisms. The unique characteristic that differentiates miRNAs from siRNAs is the ability to bind to imperfectly matched target mRNAs and inhibit translation. Thus, a single miRNA sequence may be able to silence numerous target genes that are involved in the same functional event at the same time [30] . Several miRNAs are known to drive tumorigenesis at the initiation stage and to induce invasive activity at the metastatic stage by regulation of distinct targets, as with miR-200 and miR-9 in the development of some breast cancers [31] , [32] . In this report, we found that miR-135b was overexpressed in lung cancer cells, and that miR-135b acted as an oncogenic miRNA that promoted tumour growth and cellular invasiveness and metastasis in lung cancer, enforcing its oncogenic function through the repression of multiple key components of a Hippo pathway network along with the tumour suppressor LZTS1 ( Fig. 8 ). 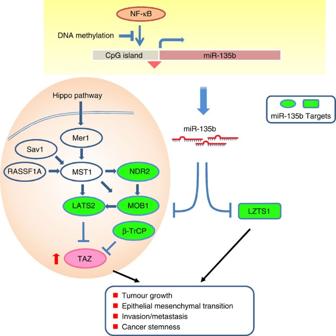Figure 8: A schematic model of regulation of lung cancer invasion and metastasis by miR-135b regulatory axis. The expression level of miR-135b is regulated by DNA methylation and NF-κB activity. Once miR-135b is upregulated, it suppresses downstream target genes such as LZTS1 and Hippo pathways, therefore promotes tumor growth, EMT, invasion/metastasis and cancer stemness. Figure 8: A schematic model of regulation of lung cancer invasion and metastasis by miR-135b regulatory axis. The expression level of miR-135b is regulated by DNA methylation and NF-κB activity. Once miR-135b is upregulated, it suppresses downstream target genes such as LZTS1 and Hippo pathways, therefore promotes tumor growth, EMT, invasion/metastasis and cancer stemness. Full size image Previous evidence has indicated that miR-135b is overexpressed in colon [33] , [34] , breast [17] and prostate [35] cancers, which strongly suggests a general role in different types of cancers. The ability of miR-135b to target multiple tumour suppressors indicates an indiscriminate ability to promote tumour progression and metastasis. Other researchers have found that miR-135b may also contribute to angiogenesis in anaplastic large-cell lymphoma [19] , implying that it has a central role in regulating several signalling pathways, thereby confirming its participation in multifarious processes during cancer development. A miR-135b antagomir (Antago-135), which is able to functionally suppress miR-135b, effectively reduced metastasis and tumour burden, which suggests the potential for the development of miR-135b antagonists for lung cancer therapy. A reduced expression of LZTS1 has been reported to correlate with poor clinical outcomes in bladder [36] , breast [37] , ovarian [38] and lung [39] , [40] cancers, and the tumour suppressor function of LZTS1 has been reported to mainly focus on reducing cell growth [41] . In the current study, we demonstrated a new function of LZTS1 in suppressing the migratory and invasive activity of tumour cells in lung cancer. We found that LZTS1 expression in tumour specimens was predictive of overall survival of NSCLC patients. In addition, LZTS1 was shown to repress the mRNA expression of Slug and Snail in MDA-MB 231 breast cancer cells [42] . Our results also showed that in LZTS1 overexpressed CL1-5 cells, the epithelial-mesenchymal-transition (EMT) regulator of Slug protein expression was suppressed, while knockdown of LZTS1 in CL1-0 cells upregulated the Slug expression ( Supplementary Fig. S9b ). Consistent with the finding that miR-135b could modulate the EMT marker, our results further support that miR-135b may control cancer invasion and metastasis through downregulating LZTS1 in lung cancer cells. We further identified a series of miR-135b target genes that functioned as tumour suppressors and belonged to a Hippo signalling pathway [28] . The mammalian Hippo pathway is mainly composed of a kinase cascade that includes MST1/2, LATS1/2, MOB1a/b and Sav1, which phosphorylates the transcriptional coactivator TAZ/YAP (refs 43 , 44 ). Phospho-TAZ protein retained in the cytoplasm is recognized by SCF β-TRCP -mediated degradation [43] . NDR1/2 shares a similar NDR domain with LATS1/2 and is phosphorylated by MST1/2 and MOB1, indicating that it may have an extended role in Hippo tumour suppressor pathways [45] . The Hippo pathway prevents overgrowth of organs and it has also recently been shown to suppress tumour growth by inhibiting TAZ (refs 46 , 47 ). Our results showed that miR-135b affected Hippo-related pathways by downregulating the levels of LATS2, NDR2, MOB1b and β-TRCP proteins. We detected variations in the downregulation levels of Hippo components in different cell lines ( Supplementary Fig. S12 ), indicating that these proteins were not coincidentally regulated by miR-135b. However, the expression levels of TAZ in lung cancer cell lines were consistently correlated with miR-135b ( Fig. 5c–e , and Supplementary Fig. S12 ). In some cases, TAZ/YAP has been shown to not be influenced by LATS2 in specific cell types [43] , however, the N-terminal phosphodegron of TAZ has been shown to be phosphorylated by GSK-3β and mediated by β-TrCP in a LATS2-independent manner [48] . It is worth noting that several reports and our results suggest that TAZ contributes to anchorage-independent growth and EMT in immortalized mammalian cells by driving the activation of a set of genes ( Supplementary Fig. S14 ) [26] . Thus, miR-135b may be able to affect functions similar to those regulated by TAZ ( Fig. 2 , and Supplementary Figs S3, S13 ). Namely, miR-135b may participate in the Hippo pathway, potentially presiding over limitless growth of tumours by stabilizing the TAZ/YAP protein via the regulation of a variety of different targets. miR-135b has also been reported to induce Wnt signalling pathway by the suppression of APC in colorectal cancers [16] , and the Hippo pathway has been reported to inhibit the Wnt pathway during heart development [49] . This crosstalk has also been described in cancer cells when the Hippo pathway retains β-catenin in the cytoplasm through a physical interaction between phosphorylated TAZ/YAP and β-catenin [50] , [51] . Our results suggest that the upregulation of miR-135b in lung cancer may antagonize the Hippo pathway and inhibit the Wnt/β-catenin pathway through direct APC and β-TrCP suppression. Thus, the finding that miR-135b can modulate multiple oncogenic pathways may make it a novel therapeutic target for cancers. Previous studies have shown that miRNAs can be epigenetically regulated and thereby contribute to metastatic processes [52] . Our results showed that the CpG islands on the miR-135b promoter region were highly methylated in low-invasive cancer cells, and that a DNA demethylating agent could increase miR-135b expression. A TNF-α-stimulated NF-κB signalling cascade synergistically acted with DNA demethylation to further elevate miR-135b expression. Quantitative pyrosequencing analysis revealed that the degree of methylation of the putative NF-κB binding sites on the miR-135b promoter was inversely related to the levels of miR-135b expression. Therefore, it appears that DNA methylation may prevent NF-κB from binding to the miR-135b promoter. It has been postulated that inflammation is strongly correlated with cancer progression, because sustained cytokine activity (for example, TNF-α and IL-6) continually activates transcription factors (AP-1, NF-κB and STAT3) and contributes to tumorigenesis and metastasis [53] , [54] , and miR-135b levels have been found to be significantly elevated in chronic colitis-related colon cancers [55] . Our study provides further evidence to support the notion that microenvironment stimulants, such as inflammatory cytokines, are exploited by cancer cells so that endogenous epigenetic mechanisms acquire metastatic ability through modulation of miRNA expression. In summary, we demonstrate a novel dual-regulatory mechanism consisting of an epigenetic factor and inflammatory stimulation that synergistically activated oncogenic miR-135b expression. Functional studies indicated that the modulation of miR-135b promoted cancer invasion and metastasis via downregulation of multiple targets in the Hippo pathway and of the tumour suppressor LZTS1. The finding that the dysregulation of miR-135b was involved in lung cancer progression indicates that a miR-135b antagomir may have a therapeutic potential for cancer treatment. Cell culture and antibodies The lung cancer cell lines CL1-0, CL1-1, CL1-5 and CL1-5-F4 were derived from in vitro transwell and in vivo metastasis selection as previously described [56] . The A549, HOP-62, H441 and CL141 cells and melanoma cell line UACC-257 were maintained in RPMI supplemented with 10% fetal bovine serum. The H1299 and HEK-293 cells were maintained in DMEM with 10% fetal bovine serum. The primary antibodies used for immunoblot analysis and immunohistochemical staining were mouse anti-LZTS1 (Abnova, Taipei, Taiwan), mouse anti-HA antibody (Covance Inc., CA, USA), rabbit anti-LATS2 (Bethyl Laboratories, Inc., Cambridge, UK), rabbit anti-βTrCP (Cell Signaling Technology, Inc., MA, USA), rabbit anti-NDR2 (Santa Cruz Biotechnology, CA, USA), rabbit anti-TAZ (Cell Signaling Technology), and mouse anti-β-actin antibody (Santa Cruz Biotechnology). Cells were seeded in 100-mm dishes at a concentration of 1 × 10 5 for treatment with 5-aza-2′-CdR (R&D Systems Inc., MN, USA) for 96 h. For TNF-α (PeproTech, Rocky Hill, NJ) stimulation, 1 × 10 6 cells were seeded in 60-mm dishes for 24 h and treated with different amounts of TNF-α for 6 h. Lentiviral vector transduction Pre-miR-135b-encoding sequences and LZTS1-encoding sequences were subcloned into the pLKO-AS2.neo vector (obtained from the National RNAi Core Facility in Academia Sinica, Taipei, Taiwan), and lentiviral vectors were prepared in accordance with standard protocols. CL1-0, UACC-257 and A549 cells were infected by lentiviruses with different multiplicities of infection in medium containing polybrene (8 μg ml −1 ). One day after infection, the cells were treated with G418 to derive a pool of neomycin-resistant clones. Bisulfite sequencing and qMS-PCR For the bisulfite sequencing, 1 μg of genomic DNA was treated with sodium bisulfite as describe in the manual (Zymo Research, Orange, CA). The bisulfite-treated DNA was desalted and eluted in 40 μl of elution buffer. Next, 2 μl of DNA was amplified with the forward primer mir-135-BF 5′-GTGTGTAAATGTTTGTATATGTGTG-3′ and the reverse primer mir-135-BR 5′-AACTTTCAAATAAATACCTAAACCC-3′. The PCR products were ligated into the TA cloning vector (RBC Bioscience, Taipei, Taiwan) and analysed to determine the DNA sequence. For qMS-PCR, 1 μg of genomic DNA was converted with an EZ DNA methylation kit (Zymo Research). Modified DNA was then subjected to real-time qMS-PCR as previously described [57] . The primers targeting the miR-135b promoter were as follows: 135b-M2F: 5′-TCGTTTCGTTTTCGTTAGTTTTTTC-3′, 135b-M2R: 5′-GATACCGAAAAACCCCCTCGTA-3′, 135b-U2F: 5′-TGTTTTGTTTTTGTTAGTTTTTTTGA-3′ and 135b-U2R: 5′-CCAATACCAAAAAACCCCCTCATA-3′. Quantitative PCR analysis Total RNA was isolated using TRIZOL reagent (Invitrogen, Carlsbad, CA) according to the standard protocol. The mature miR-135b and endogenous control U6B were analysed using TaqMan MicroRNA Assays (Applied Biosystems, Foster City, CA). Briefly, 30 ng of total RNA was reverse-transcribed via SuperScript-III reverse transcriptase (Invitrogen, Carlsbad, CA). The cDNA was amplified with a TaqMan 2 × Universal Master Mix (Applied Biosystems), and miRNA-specific real-time PCR was performed using an ABI 7500 real-time PCR system. Luciferase reporter assay One day before transfection, CL1-0 cells were seeded in 12-well plates at a concentration of 2.5 × 10 4 per well. Next, 100 or 200 ng of pCIneo vector or miR-135b plasmid was co-transfected with 50 ng of pGL3-target gene-3′-UTR. The Renilla luciferase plasmid (phRL-TK, Promega, Madison, WI) was co-transfected as a transfection control. Cells were lysed 36 h after transfection, and luciferase activity was measured using a Dual-Luciferase system (Promega, Madison, WI) according to the manufacturer’s protocol. Invasion and migration assay Transwell chambers (8-μm pore size; BD Falcon, Franklin Lakes, NJ) were coated with the appropriate amount of 5 μg ml −1 Matrigel (BD Biosciences, San Jose, CA). Next, 2.5 × 10 4 cells were suspended in 10% NuSerum-containing media (Gibco BRL, Grand Island, NY, USA), seeded in the chamber and cultured for 20 h. Cells that invaded the chamber from top to bottom were fixed with methanol and stained with a 50-μg ml −1 solution of propidium iodine (Sigma-Aldrich, St. Louis, MO). The propidium iodine-positive signal was quantified using the Analytical Imaging Station software package. Each sample was assayed in triplicate. For the migration assay, culture inserts (Ibidi, Munich, Germany) were inserted into 60-mm dishes. Next, 70 μl of the cell suspensions were seeded in each culture insert well at a concentration of 2.5 × 10 4 (CL1-0) or 3 × 10 4 (CL1-5-F4 and UACC-257) cells per ml. The culture inserts were removed 24 h later to leave a gap of ~ 500 μm. Cell migration was observed at different time points, and the number of cells that migrated into the gap was calculated. In vivo animal models Animals were housed in a specific-pathogen-free environment in the animal facility of the Institute of Biomedical Sciences, Academia Sinica. All experimental procedures were in compliance with the Academia Sinica IACUC and Council of Agriculture Guidebook for the Care and Use of Laboratory Animals. For intravenous injections of the tumour cells, 1 × 10 6 cells were suspended in 0.1 ml of phosphate-buffered saline (PBS) and injected into the lateral tail vein of SCID mice (10 mice per group). At 8 weeks after injection, all mice were killed, and lung surface tumour foci were counted. For the subcutaneous tumour growth assay, 1 × 10 6 CL1-0 cells or 2 × 10 5 H441 cells were subcutaneously injected in 0.1 ml of PBS into male nude mice ( n =8 per group) and allowed to grow for 35 days to reach a volume of 50–200 mm 3 . Control antagomir (Scramble) or anti-miR-135b antagomir (antago-135) was intravenously injected at a concentration of 10 μM in 0.1 ml of PBS 4 days after the cells were implanted. For the orthotopic tumour implantation assays, lentivirus-infected CL1-0/vector orCL1-0/miR-135b-overexpressing cells (10 5 cells in 20 μl of PBS containing 10 ng of Matrigel) were injected into the pleural cavity of 6-week-old SCID mice ( n =10 per group). The mice were killed by carbon dioxide anaesthesia 28 days after implantation and the lungs were removed and fixed in 10% formalin. The lung nodules were counted by gross and microscopic examination. The number of mice used for the experiments ( n =10) was based on the goal of having 98% power to detect a two-fold between-group difference in the number of modules at P <0.05. Clinical lung cancer samples and immunohistochemistry Frozen lung cancer specimens from 112 consecutive patients who underwent surgical resection of NSCLC at the Taichung Veterans General Hospital were analysed for the expression of miR-135b. None of the patients had received adjuvant chemotherapy. miRNA expression profiling was performed using a TaqMan MicroRNA Assay Kit (Applied Biosystems, Foster City, CA) and an ABI PRISM 7900 real-time PCR System. miR-135b expression was quantified in relation to the expression of small nuclear U6 RNA. In addition, samples from 147 NSCLC patients who underwent surgical resection at the National Taiwan University Hospital were analysed for the expressions of LZTS1, LATS2 and TAZ. Sections were fixed in formalin and embedded in paraffin. The primary antibodies against LZTS1 (anti-FEZ), LATS2 and TAZ were obtained from BD Biosciences (San Jose, CA), Bethyl Laboratories Inc. and Cell Signaling, respectively. PBS without primary antibodies was applied as the negative control. The immunohistochemistry results were scored and classified into two groups according to the average staining intensity and area. Group 1 corresponded to a positive staining of <50% of the tissue section, and group 2 corresponded to a positive staining of >50% of the tissue section. The immunostaining results were assessed and scored independently by two pathologists. Chromatin immunoprecipitation CL1-0 and H1299 cells were fixed with 1% formaldehyde for 10 min and blocked by 125 mM glycine for 5 min. The cells were resuspended in cell lysis buffer (5 mM HEPES, 85 mM KCl, 0.5% Triton X-100, 1 mM DTT, 1 mM PMSF, pH 8.0), followed by nucleic lysis buffer (50 mM Tris-HCl, 10 mM EDTA, 1% SDS, 1 mM DTT and protease inhibitor (Roche Applied Science, Mannheim, Germany)). The cell lysate was sonicated with six 10-s pulses and clarified by centrifugation for 10 min. The supernatant was diluted with 40 μl of protein G beads for 30 min at 4 °C to pre-clear the solution. Immunoprecipitation with anti-RelA (Abcam, Cambridge, UK) was performed at 4 °C overnight. DNA–protein complexes were then incubated with protein G agarose beads at 4 °C with constant rotation for 2 h. Following immunoprecipitation, the beads were washed with a low-salt wash buffer, a high-salt wash buffer, a LiCl wash buffer and, finally, a TE buffer. The immunoprecipitated complexes were eluted in a buffer containing 10 mM Tris pH 8.0, 300 mM NaCl, 5 mM EDTA and 0.5% SDS at room temperature for 6 h. The samples were then treated with proteinase K for 1 h, followed by RNAse A for 1 h. Next, the DNA was purified by phenol/chloroform extraction. The DNA was submitted for PCR amplification with primers specific to the miR-135b promoter region: the forward primer was 5′-GAGTGGCGGGGGTAGGAGGG-3′, and the reverse primer was 5′-GCAACTTCGCGCCTAAGCGC-3′. Statistical analysis Data are presented as the mean±s.d., The differences between two groups were assessed using the Student’s t -test, and the Kaplan–Meier method was used to estimate overall survival. Differences in survival between two groups were analysed using the log-rank test. Multivariate Cox proportional hazard regression analysis with stepwise selection was used to evaluate independent prognostic factors associated with patient survival, and the expression of miR-135b, age, gender, tumour stage and histology were used as covariates. All analyses were performed with SAS version 9.1 software (SAS Institute Inc.). Two-tailed tests were used, and P -values<0.05 were considered to indicate statistical significance. How to cite this article: Lin, C. -W. et al . MicroRNA-135b promotes lung cancer metastasis by regulating multiple targets in the Hippo pathway and LZTS1. Nat. Commun. 4:1877 doi: 10.1038/ncomms2876 (2013).